Radiation-resistant metal-organic framework enables efficient separation of krypton fission gas from spent nuclear fuel Capture and storage of volatile radionuclides that result from processing of used nuclear fuel is a major challenge. Solid adsorbents, in particular ultra-microporous metal-organic frameworks, could be effective in capturing these volatile radionuclides, including 85 Kr. However, metal-organic frameworks are found to have higher affinity for xenon than for krypton, and have comparable affinity for Kr and N 2 . Also, the adsorbent needs to have high radiation stability. To address these challenges, here we evaluate a series of ultra-microporous metal-organic frameworks, SIFSIX-3-M (M = Zn, Cu, Ni, Co, or Fe) for their capability in 85 Kr separation and storage using a two-bed breakthrough method. These materials were found to have higher Kr/N 2 selectivity than current benchmark materials, which leads to a notable decrease in the nuclear waste volume. The materials were systematically studied for gamma and beta irradiation stability, and SIFSIX-3-Cu is found to be the most radiation resistant. Nuclear energy is an emission free, high-energy density source with minimal land use. However, any future expansion of civilian nuclear power will most likely require efficient management of used nuclear fuel (UNF). UNF processing minimizes radioactive waste, but the release of volatile radionuclides is a significant challenge. The nature of the volatile radionuclides depends on the reprocessing procedure and generally consists of a mixture of noble gases (predominantly 85 Kr, which β or βγ decays to stable 85 Rb with t 1/2 = 10.8 years, along with Xe), and species containing 129 I [1] , [2] , [3] , [4] , [5] . The current reprocessing technologies can capture other volatile radionuclides with relative ease, but an efficient system to capture (and store) 85 Kr needs to be in place. While methods such as cryogenic distillation and fluorocarbon based absorption have been proposed and tested, they are expensive and require complex engineering control. Solid-state adsorbents, in particular porous metal-organic frameworks (MOFs), could be better alternatives to capture these volatile radionuclides including 85 Kr. Physisorption-based adsorption and storage is deemed an energy-efficient process that can be operated at near-ambient conditions and is easier to integrate into current engineering setups. Several traditional adsorbents such as zeolites and activated carbon have been tested, but were found to have low capacity and selectivity (over Xe and other competing gases). MOFs are known for their versatile architecture and functionalized pore surface and have shown promise for gas sorption and separation [1] , [6] , [7] , [8] , [9] , [10] , [11] , [12] , [13] , [14] , [15] , [16] . However, as Xe is considerably more polarizable than Kr, porous materials such as MOFs are generally more selective toward Xe over Kr due to stronger van der Waals interactions, which causes further engineering challenges as the Xe will lead to reduced Kr adsorption [2] , [7] , [15] , [17] , [18] , [19] . To avoid this, we recently reported a proof-of-concept study where a dual-bed system, fitted in series, was utilized to separate and store Kr [20] . The gas stream (known as off-gas, 400 ppm of Xe and 40 ppm of Kr mixed with air, which are the typical concentrations of the off-gas in a reprocessing plant) is first directed through a Xe selective adsorbent bed to remove the Xe, followed by removal of Kr in the second bed using the same or another adsorbent material. In the absence of the competing Xe in the second bed, the adsorbent is expected to have enhanced Kr storage capacity, even when using identical adsorbent material (which is the modality used in this paper). The enhancement and the total Kr uptake depend on the selectivity for Kr over competing gases (e.g., N 2 , O 2 ). The stored gas in the second bed has a high Kr, low Xe feature, so the second bed can be fluidized and/or regenerated (with temperature controlled desorption) with such characteristics in mind. The MOFs in both the first bed and the second bed should be sufficiently radiation resistant to beta and gamma radiations as 85 Kr flows pass or stores in them. Only a few MOFs have been studied for their radiation stability [20] , [21] . Lee et al. reported the potential of three MOFs (MIL-100(Fe), MIL-101(Cr), and UiO-66(Zr)) for Xe/Kr separation [22] . The study showed that UiO-66(Zr) is the most promising adsorbent among the three candidates; however, the radiation stability of UiO-66(Zr) has been performed under low radiation dose of only 2 kGy which is not relevant to the practical Xe/Kr separation at nuclear reprocessing plants. In our continuous search for materials with high Kr adsorption capacity and selectivity, we synthesized, measured and analyzed the SIFSIX-3-M series (M = Zn, Cu, Ni, Co, Fe) of MOFs [7] , [23] , [24] , [25] . SIFSIX-3-M is a class of isoreticular hybrid ultra-microporous materials (HUMs) based on saturated metal centers (SMCs) and SiF 6 −2 pillars [26] , [27] . SIFSIX-3-M can be tuned for Kr separation by substituting different metal centers including Zn [27] , [28] , Co [29] , Cu [30] , Ni [29] , or Fe [8] . SIFSIX-3-M materials are known for their very low affinity toward N 2 and for exceptional performance in selectively removing CO 2 from air, which makes them great candidates for two-bed breakthrough setup. In this study, two columns were filled by adsorbent material that has a preferential adsorption of gases Xe, CO 2 > Kr > N 2 and O 2 . The Xe and CO 2 gases will be selectively adsorbed over the rest of gases in the first bed while the Kr will be preferentially adsorbed over the N 2 and O 2 in the second bed. The advantage of this method is that we can separate the radioactive 85 Kr into a high purity gas. The presence of other gases mixed with 85 Kr would otherwise increase the waste volume to be disposed and therefore increase the cost of the UNF reprocessing (Fig. 1 ). Fig. 1: Schematic representation of the two-bed breakthrough setup. a Illustration of the two-bed technique for removal of radioactive Kr from nuclear reprocessing plants using SIFSIX-3-Cu. b Each two squares in the bed 1 and bed 2 represent two channels of SIFSIX-3-Cu structure. Atom colors: C = gray, H = white, N = light blue, F = green, Si = light brown, Cu = orange, O = red, Xe = violet, Kr = pink. Full size image Radiation stability study The MOF materials were exposed to gamma radiation ( 60 Co source) from 0 to 200 kGy and the stability of the materials was monitored by powder X-ray diffraction (PXRD) to confirm the retention of their crystallinity after γ irradiation (see Methods section for experimental details) and β irradiation. The near equivalence in radiation damage tolerance dose between 85 Kr β and 60 Co γ-rays was well established, for example “no significant difference in the decomposition yield was observed” in fluorocarbons exposed to beta and gamma radiation of the same dose [31] . Quantitative analyses of the PXRD data using the Rietveld and Pawley fitting methods were performed to compare the as-synthesized structures with the irradiated structures (Supplementary Figs. 3 – 17 ). As shown in Figs. 2 and 3 and Supplementary Figs. 3 and 4 , the Zn and Ni analogs are unstable and show phase change at 1 kGy. SIFSIX-3-Fe maintained its crystallinity at 1 kGy. Further irradiation of SIFSIX-3-Fe to 3 and 10 kGy leads to new unknown phases as shown in Supplementary Figs. 4 – 8 . The new phase is a mixture of a 1D structure with water coordinated to Fe (Fig. 2 ) and another unknown phase. The original structure of SIFSIX-3-Fe is strongly distorted and almost vanished. The SIFSIX-3-Co structure was stable up to 10 kGy before it undergoes phase change (Supplementary Figs. 9 – 12 ). From the PXRD pattern of irradiated MOF at 3 kGy, higher peak intensity for the (110) peak at 17.65° was observed which may be attributed to spinning of fluorine atoms into the (110) plane (Supplementary Fig. 11 ). Based on these results the crystal structure of SIFSIX-3-Co remains unaltered under 3 kGy radiation. After 10 kGy radiation, the crystal structure is altered and presents the original SIFSIX-3-Co structure as well as another unknown phase. The unit cell and space group are determined from the unknown phase peak positions (Supplementary Fig. 12 ) to be tetragonal (4/m) with lattice parameters a = 16.086 Å and c = 12.952 Å, which does not exist in the CCDC database [32] . Fig. 2: Illustration of impact of irradiation on SIFSIX-3-M materials. The SIFSIX-3-M (M = Zn, Co, Ni, Fe) structures decompose to 1D, 2D or many other possible phases up on radiation exposure. The SIFSIX-3-Cu is stable and maintains its original crystal structure up to 50 kGy dose in beta or gamma radiation. Atom colors: C = gray, H = white, N = light blue, F = green, Si = light brown, Cu = orange, M (Ni, Co, Fe, Zn) = cyan, O = red. Full size image Fig. 3: Powder X-ray diffraction patterns of irradiated and simulated SIFSIX-3-M structures. a gamma-irradiated SIFSIX-3-Zn, b gamma-irradiated SIFSIX-3-Ni, c gamma-irradiated SIFSIX-3-Fe, d gamma-irradiated SIFSIX-3-Co, and e SIFSIX-3-Cu and f activated SIFSIX-3-Cu structure after 50 kGy beta irradiation. Full size image SIFSIX-3-Cu was the most stable MOF (Supplementary Figs. 13 – 17 ) and it maintained its crystallinity up to 50 kGy γ irradiation. According to Cambridge Structural Database (CSD) [33] , Cu tends to bond with N donor ligand more readily compared with Co, Fe, Zn, and Ni. The Cu–N bonds are stronger than those of other M–N analogs. This is supported by shorter Cu–N bond distance of 1.9 Å in the SIFSIX-3-Cu compared with the other the M–N analogs (2.1 Å). Also, it was reported that the SIFSIX-3-Cu has a slightly smaller unit cell of 378 Å 3 versus 388 Å 3 (SIFSIX-3-Zn), where the authors attributed this observation to the relatively stronger bonding between the Cu(II) and the pyrazine [30] . Therefore, M–N bond strength could be the main factor behind the stability of SIFSIX-3-Cu framework which reaches up to 50 kGy, while other materials demonstrate much lower stability that reaches to maximum 10 kGy (in case of Co). For this class of the isoreticular SIFSIX-3-M structures, it was reported that the change in metal center or the environment around it could lead to different properties of the MOF material [8] , [21] , [29] , [30] , [34] . The beta radiation stability of the SIFSIX-3-Cu was evaluated by irradiating the activated sample with 1.5 MeV electrons beam at a dose rate of 50 kGy/h and comparing its PXRD pattern with the simulated SIFSIX-3-Cu pattern. Figure 3f showed that the activated SIFSIX-3-Cu sample is stable after 50 kGy beta irradiation. 85 Kr concentration is reported to be 1130–1800 TBq/Mg (3510–48,600 Ci/Mg) of spent fuel [35] . 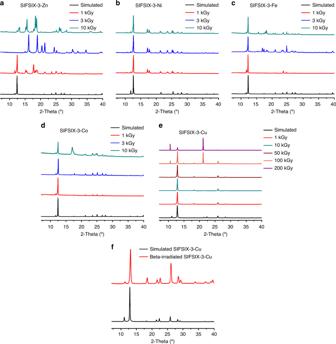Fig. 3: Powder X-ray diffraction patterns of irradiated and simulated SIFSIX-3-M structures. agamma-irradiated SIFSIX-3-Zn,bgamma-irradiated SIFSIX-3-Ni,cgamma-irradiated SIFSIX-3-Fe,dgamma-irradiated SIFSIX-3-Co, andeSIFSIX-3-Cu andfactivated SIFSIX-3-Cu structure after 50 kGy beta irradiation. Based on these concentrations, the radiation dose rate to 1 g SIFSIX-3-Cu from absorbing all the 85 Kr in 1 g of spent nuclear fuel was calculated (see Supplementary Note 3 ). According to the obtained results from both beta and gamma irradiation experiments, SIFSIX-3-Cu is radiation resistant up to 50 kGy. Hence, 1 g of SIFSIX-3-Cu can separate 85 Kr effectively from 2674 g of spent nuclear fuel (130 TBq/Mg case) or 188 g spent nuclear fuel (1800 TBq/Mg case), without any crystal structure damage, if keeping all the 85 Kr inside for 1 h. Single-component gas adsorption study The single-component CO 2 , Xe, Kr, N 2 , and O 2 adsorption isotherms of SIFSIX-3-Cu at 298 K (Fig. 4a ) showed a preferential adsorption of CO 2 and Xe over Kr which will allow CO 2 and Xe capture in the first bed, and a high Kr/N 2 selectivity which facilitates the capture of the 85 Kr in the second bed. Fig. 4: Gas adsorption properties and binding sites. a Single-component CO 2 , Xe, Kr, N 2 , and O 2 adsorption isotherms at 298 K for SIFSIX-3-Cu. Molecular illustration of the most favorable binding site for b Xe and c Kr in SIFSIX-3-Cu (top view) as determined from simulated annealing calculations. Atom colors: C = cyan, H = white, N = blue, F = green, Si = yellow, Cu = gold, Xe = violet, Kr = pink. Full size image Modeling study As revealed through modeling studies, the larger atomic radius for Xe provided for a better fit within the square pores as well as the region enclosed by four neighboring SiF 6 2– pillars in the material (Fig. 4b, c and Supplementary Figs. 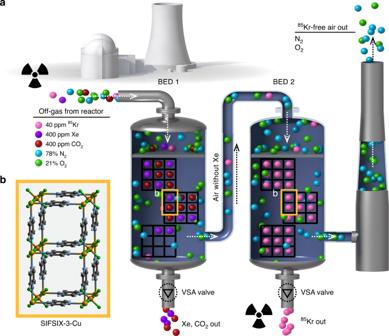23 and 24 ). 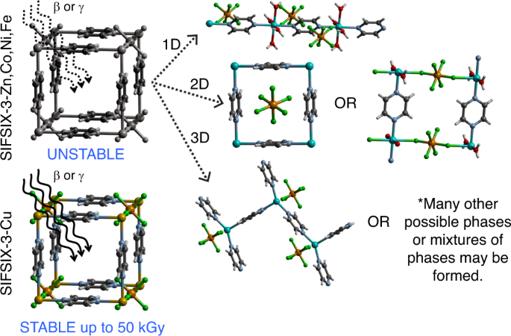Fig. 1: Schematic representation of the two-bed breakthrough setup. aIllustration of the two-bed technique for removal of radioactive Kr from nuclear reprocessing plants using SIFSIX-3-Cu.bEach two squares in the bed 1 and bed 2 represent two channels of SIFSIX-3-Cu structure. Atom colors: C = gray, H = white, N = light blue, F = green, Si = light brown, Cu = orange, O = red, Xe = violet, Kr = pink. Fig. 2: Illustration of impact of irradiation on SIFSIX-3-M materials. The SIFSIX-3-M (M = Zn, Co, Ni, Fe) structures decompose to 1D, 2D or many other possible phases up on radiation exposure. The SIFSIX-3-Cu is stable and maintains its original crystal structure up to 50 kGy dose in beta or gamma radiation. Atom colors: C = gray, H = white, N = light blue, F = green, Si = light brown, Cu = orange, M (Ni, Co, Fe, Zn) = cyan, O = red. Furthermore, density functional theory (DFT) calculations confirm that SIFSIX-3-Cu is selective for CO 2 and Xe over Kr, and Kr over N 2 and O 2 on the basis of the DFT calculated adsorption energies in the material (see Supplementary Note 5 and Supplementary Table 1 ). Two-bed breakthrough adsorption study We ran the two-bed breakthrough experiments, where both beds use SIFSIX-3-Cu, because of its high radiation stability (Fig. 3e ). First, a single-bed test was performed on SIFSIX-3-Cu (Fig. 5a, b) in order to show the ability of SIFSIX-3-Cu for separation of Kr gas from N 2 and O 2 . Second, single-bed experiments were run for the simulated off-gas containing 400 ppm Xe and 40 ppm Kr balanced with dry air, revealing the time needed for each gas to break through from the first bed under the conditions of simulated off-gas stream. Accordingly, this information informed us of when to switch on the second bed in the two-bed system before Xe and CO 2 start to break through (see Fig. 1 , Supplementary Note 6 and Supplementary Scheme 1 ). The single-bed breakthrough experiments for 1000 ppm Kr balanced with dry air revealed that SIFSIX-3-Cu can selectively adsorb Kr over N 2 and O 2 as shown in Fig. 5 and Table 1 . Fig. 5: Breakthrough curves for SIFSIX-3-Cu. a Single-bed breakthrough experiment using 1000 ppm Kr balanced with dry air. b Single-bed breakthrough experiment using 400 ppm Xe and 40 ppm Kr balanced with dry air. c Two-bed breakthrough experiment using 400 ppm Xe and 40 ppm Kr balanced with dry air. d schematic demonstration of the concept of the two-bed technique for the 85 Kr removal from the UNF. Full size image Table 1 Xe and Kr separation performance parameters for SIFSIX-3-Cu at 298 K and 1 bar. Full size table Based on the single-column experiment, SIFSIX-3-Cu can selectively separate Xe from gas mixture 1 consisting of 400 ppm Xe, 40 ppm Kr balanced with dry air. The column breakthrough experiment suggests that Xe breakthrough occurs at t 1 finish = 29 min, thus by connecting a second bed loaded with adsorbent material before this time, we will be able to capture the Kr in the second bed before the Xe breaks through the first bed (see Fig. 5 ). We note that t 1 finish certainly depends on the size and geometric design of the first bed (which can be fluidized [36] ), i.e., it is not just a material property. The two-column breakthrough system consists of two adsorption beds in series that were packed with 1 g of SIFISIX-3-Cu in each bed. 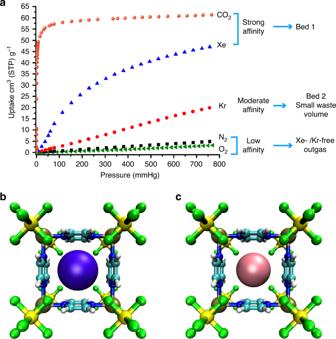Fig. 4: Gas adsorption properties and binding sites. aSingle-component CO2, Xe, Kr, N2, and O2adsorption isotherms at 298 K for SIFSIX-3-Cu. Molecular illustration of the most favorable binding site forbXe andcKr in SIFSIX-3-Cu (top view) as determined from simulated annealing calculations. Atom colors: C = cyan, H = white, N = blue, F = green, Si = yellow, Cu = gold, Xe = violet, Kr = pink. 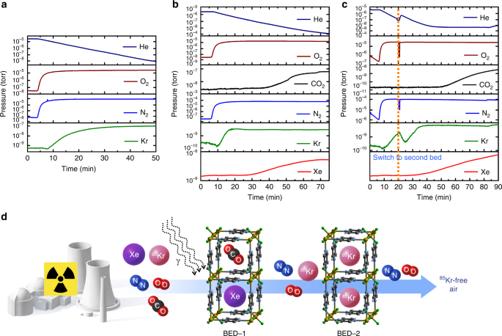Fig. 5: Breakthrough curves for SIFSIX-3-Cu. aSingle-bed breakthrough experiment using 1000 ppm Kr balanced with dry air.bSingle-bed breakthrough experiment using 400 ppm Xe and 40 ppm Kr balanced with dry air.cTwo-bed breakthrough experiment using 400 ppm Xe and 40 ppm Kr balanced with dry air.dschematic demonstration of the concept of the two-bed technique for the85Kr removal from the UNF. The adsorbent beds were purged with He and then a gas mixture containing 400 ppm Xe and 40 ppm Kr balanced with dry air at a total pressure of 1 bar was introduced to the first bed (with the second bed bypassed). Breakthrough curves indicate that the Xe gas and CO 2 were retained by the first bed, leaving 40 ppm Kr balanced with dry air at the outlet. At time t 2 start = 18 min, the second bed was enabled, thus flowing gas from the first bed to the second. Gas analysis shows that Kr concentration drops as it is adsorbed into the second bed, and fully breaks through again at t 2 finish = around 30 min. In practice the feed gas would be directed to a new bed, while the Kr loaded bed is regenerated. It is important to note that the adsorbent material can capture Kr gas over the competing gases that could increase the waste volume. The benchmark materials, SBMOF-1 [37] , Ni-MOF-74 [38] , and Ag mordenite [39] , showed remarkable performance for Xe/Kr separation, however, they are not suitable for 85 Kr separation from spent fuel using the two-bed technique. Ni-MOF-74 [38] and Ag mordenite [39] were found to have poor Kr/N 2 selectivity (Supplementary Figs. 21 and 30 ), while, SBMOF-1 [37] showed low Kr/CO 2 which prohibit the separation of the Kr in pure form (Supplementary Fig. 22 ). As shown in Fig. 5 and Table 1 , SIFISIX-3-Cu showed a great potential for Kr removal from simulated UNF off-gas using the two-bed system. The calculated capacity of the adsorbed Xe in first bed by SIFSIX-3-Cu at equilibrium was found to be 6.74 mmol/kg while the capacity of the Kr captured in second bed is 0.15 mmol/kg. This system is a feasible and efficient way to separate and capture Xe and Kr at ambient conditions. This further demonstrates that once the competing gas, Xe, is removed in the first bed using SIFSIX-3-Cu, the Kr removal efficiency was increased significantly, which can lead to a notable decrease in the waste volume at the UNF reprocessing plant. In summary, we evaluated the performance of a family of ultra-microporous pillared square lattices, SIFSIX-3-M (M = Fe, Co, Ni, Cu, Zn) for 85 Kr removal from used nuclear fuel. The radiation stability was examined by exposing the materials to varying levels of gamma radiation and beta radiation. SIFSIX-3-Cu is the only material in this family suitable for this application based on radiation stability up to 50 kGy for both beta and gamma radiations. The choice of the right material for the 85 Kr separation from nuclear reprocessing plants is based on several criteria: (1) Preferential adsorption of Xe and CO 2 over Kr so these two gases can be separated in the first bed, and (2) Preferential adsorption of Kr over N 2 and O 2 so that Kr can be adsorbed in the second bed in more pure form with minimum waste volume. If the material fulfills these two criteria, then it should be qualified for the radiation stability. If the material does not achieve these two criteria, it is not helpful in this context to examine their radiation stability because they did not fulfill the main purpose of the Kr removal presented herein, which is the reduction of waste volume and Kr separation in more pure form with minimal amounts of other competing gases. The single-component adsorption isotherms revealed that SIFSIX-3-Cu can preferentially adsorb CO 2 and Xe over Kr, and Kr over N 2 and O 2 ; these findings have been supported by modeling. The practical use of SIFSIX-3-Cu in Kr capture and separation from nuclear fuel reprocessing off-gas was demonstrated by using a two-bed breakthrough technique at ambient conditions. SIFSIX-3-Cu successfully captures Xe in the first bed, while high purity Kr gas is captured in the second bed using the same material. We attribute the remarkable performance of SIFSIX-3-M family to the narrow pore size as well as the high polarizability of SiF 6 −2 anions. Indeed, modeling studies revealed that the adsorbate localizes between four neighboring SiF 6 2– pillars within the small pores in this class of materials. Synthesis [M(pyz) 2 SiF 6 ] (SIFSIX-3-M, M = Zn, Cu, Ni, Co, Fe) was synthesized by dissolving 10 mmol of pyrazine ligand (pyz) and 5 mmol of MSiF 6 salt in 23 mL of methanol and heating the resulting solution at 75 °C for 3 days in a stainless steel Parr autoclave [8] , [29] . SIFSIX-3-Zn and SIFSIX-3-Co afford colorless and red crystals, respectively; while SIFSIX-3-Cu, SIFSIX-3-Ni, and SIFSIX-3-Fe afford blue, pale blue, and yellow crystalline powders, respectively. All structures possess six coordinated saturated metal centers that serve as 6-connected nodes with pcu topology through four equatorial pyrazine linkers and 2 axial SiF 6 −2 anion pillars to form the 3D-pillared square-grid nets. Gamma irradiation measurements The MIT gamma irradiation facility, managed by the MIT Radiation Protection Program (RPP), houses a Gammacell 220 Excel self-shielded high dose-rate gamma ray irradiator (Supplementary Fig. 1 ) manufactured by MDS Nordion. The unit was manufactured in Canada by MDS Nordion on 13/10/2003 and contained an initial quantity of Cobalt-60 of 23,654 Curies (375.2 TBq) (Supplementary Fig. 2 ). The Co-60 sources are contained within a lead biological shield which allows for the safe use of the irradiator by trained radiation workers. The Co-60 sources are arranged in a circle allowing for a uniform dose to the materials being irradiated. The samples ae loaded in the sample irradiation chamber and lowered by elevator to the Co-60 source array. The inside dimensions of the chamber are 6.10 in (15.49 cm) diameter and 8.06 in (20.47 cm) high. The current chamber dose rate is 4235 Rads/min (42.35 Gy/min). The original chamber dose rate was 32,228 Rads/min (322.28 Gy/min). Beta irradiation measurements Experiments were performed at MIT’s High Voltage Research Laboratory (HVRL), which houses a continuous-wave Van de Graaff electron accelerator capable of producing electron kinetic energies of 1.5–3.0 MeV at beam currents of up to 30 μA. Samples were irradiated with 1.5 MeV electrons beam at a dose rate of 50 kGy/h. Powder X-ray diffraction measurements after gamma irradiation The powder X-ray diffraction (PXRD) was collected on the PANalytical X’Pert Pro using 1.8 kW sealed X-ray tube source and Cu target. In order to solve the XRD data we use high score plus program to open the data and we used Rietveld and Pawley fitting methods.